Association analysis identifies new risk loci for non-obstructive azoospermia in Chinese men Male factor infertility affects one-sixth of couples worldwide, and non-obstructive azoospermia (NOA) is one of the most severe forms. Our previous genome-wide association study (GWAS) identified three susceptibility loci for NOA in Han Chinese men. Here we test promising associations in an extended three-stage validation using 3,608 NOA cases and 5,909 controls to identify additional risk loci. We find strong evidence of three NOA susceptibility loci ( P <5.0 × 10 −8 ) at 6p21.32 (rs7194, P =3.76 × 10 −19 ), 10q25.3 (rs7099208, P =6.41 × 10 −14 ) and 6p12.2 (rs13206743, P =3.69 × 10 −8 ), as well as one locus approaching genome-wide significance at 1q42.13 (rs3000811, P =7.26 × 10 −8 ). In addition, we investigate the phenotypic effect of the related gene ( gek , orthologous to CDC42BPA ) at 1q42.13 on male fertility using a Drosophila model. These results advance our understanding of the genetic susceptibility to NOA and provide insights into its pathogenic mechanism. Infertility is one of the most frequently diagnosed diseases in reproductive health and male-related problems that account for approximately half of all infertility cases [1] , [2] . A significant proportion of male infertility is accompanied by idiopathic azoospermia, most often presenting as non-obstructive azoospermia (NOA), which occurs in ~\n1% of all adult men [3] . A few studies have reported that genetic factors including chromosome number defects, Y-chromosome microdeletions and autosomal mutations or polymorphisms in multiple biological pathways are involved in the development of NOA [4] , [5] , [6] . We recently conducted a multistage genome-wide association study (GWAS) of NOA in Han Chinese based on genotyping 587,347 single nucleotide polymorphisms (SNPs) in 981 NOA cases and 1,657 controls with a two-stage validation using 1,946 NOA cases and 4,077 controls [7] . We identified three well-replicated susceptibility loci (rs12097821 at 1p13.3 for PRMT6 , rs2477686 at 1p36.32 for PEX10 and rs10842262 at 12p12.1 for SOX5 ) [7] . Here we evaluate promising associations in an extended three-stage validation using 3,608 NOA cases and 5,909 controls, and we focus on the SNPs that have P values ranging from 10 −5 to 10 −7 in the GWA scan ( Supplementary Fig. 1 and Supplementary Data 1 ). In addition, we knocked down the genes that map to susceptibility loci that also have Drosophila homologues to investigate the phenotypic effect on male fertility. We find strong evidence of three NOA susceptibility loci ( P <5.0 × 10 −8 ) at 6p21.32 (rs7194 in HLA-DRA, P =3.76 × 10 −19 ), 10q25.3 (rs7099208 close to ABLIM1 , P =6.41 × 10 −14 ) and 6p12.2 (rs13206743 between MIR133B and IL17A , P =3.69 × 10 −8 ), as well as one locus approaching genome-wide significance (rs3000811 at 1q42.13, upstream of CDC42BPA , P =7.26 × 10 −8 ). In addition, we show the phenotypic effect of the related gene ( gek , orthologous to CDC42BPA ) on male fertility by using Drosophila as an animal model. These results advance our understanding of the susceptibility to NOA in Chinese men. Susceptibility loci of NOA in validation studies Seventy-seven SNPs met the selection criteria for the first-stage validation (Methods, Supplementary Fig. 1 and Supplementary Data 1 ). Additive models of logistic regression analyses were used to estimate the P values of association analyses. 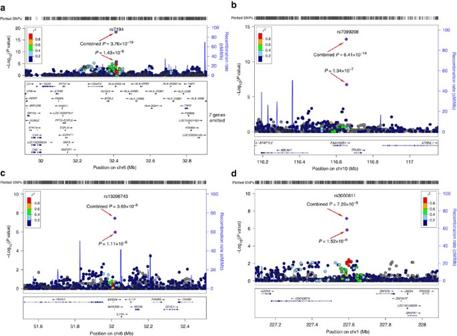Figure 1: Regional plot of the four identified lead SNPs. These SNPs are rs7194 at 6p21.32, rs7099208 at 10q25.3, rs13206743 at 6p12.2 and rs3000811 at 1q42.13. Additive models of logistic regression analyses were used to estimate thePvalues of association analyses in 981 NOA cases and 1,657 controls. The results (−log10P) are shown for SNPs in the region flanking 500 kb on either side of the marker SNPs. The marker SNPs are shown in purple, and ther2values of the rest of the SNPs are indicated by different colours. The genes within the region of interest are annotated, with arrows indicating transcription direction. For each plot, the recombination rates (rightyaxes) of the region are shown according to their chromosomal positions (xaxis). The 77 SNPs identified in the GWA scan and the three validations are shown in Table 1 , Supplementary Fig. 1 and Supplementary Data 1 . Among them, 9 SNPs (rs12023502, rs3000811, rs13206743, rs7194, rs7099208, rs4903393, rs1990264, rs4791224 and rs6055276) were consistently replicated in 1,144 NOA cases and 2,373 male controls with the same direction of significant associations as those in the GWA scan ( Table 1 and Supplementary Data 1 ). For the second-stage validation, additional 1,662 NOA cases and 2,535 male controls were genotyped to verify the significant associations of the 9 loci; 6 of the 9 loci (rs3000811, rs13206743, rs7194, rs7099208, rs1990264 and rs4791224) were consistently associated with NOA risk ( Table 1 and Supplementary Data 1 ). We then included an independent GWAS of NOA in Han Chinese [8] as the third-stage validation with 802 NOA cases and 1,001 male controls to confirm our associations. Four SNPs (rs3000811, rs7194, rs7099208 and rs13206743) were associated with NOA risk with the same direction as those in our GWA scan and the first two validations ( Table 1 , Supplementary Fig. 1 and Supplementary Data 1 ). Table 1 Association of 4 SNPs to azospermia in the GWA scan and validation studies. Full size table Combined analysis of the susceptibility loci In the combined analysis, meta-analysis was used to combine the results of GWAS scan and three validations. Three SNPs reached genome-wide significance ( P <5.0 × 10 −8 ) for NOA susceptibility in 4,589 cases and 7,566 controls; these SNPs are located at 6p12.2 (rs13206743, P combined =3.69 × 10 −8 , odds ratio (OR)=1.35), 6p21.32 (rs7194, P combined =3.76 × 10 −19 , OR=1.30) and 10q25.3 (rs7099208, P combined =6.41 × 10 −14 , OR=1.41). Another SNP (rs3000811 at 1q42.13) has a P value approaching the genome-wide significance ( P combined =7.26 × 10 −8 , OR=1.19) ( Table 1 ). After examining heterogeneity in ORs across the initial GWAS and validation stages, no significant heterogeneity was observed for the four SNPs. Stratified analyses by study regions As the subjects were collected from different regions that are geographically distant and most likely genetically differentiated, we performed stratified analyses by four study regions (Southeastern China: Nanjing and Shanghai; Central China: Wuhan; Northern China: Shenyang; and Southern China: Nanning). Similar association strengths were shown between regions in absence of significant heterogeneity for each locus ( Supplementary Table 1 ). Imputation analysis in the GWAS An imputation analysis in the GWA scan of 981 cases and 1,657 controls identified associations of SNPs with NOA risk at P ≤1.0 × 10 −5 (imputed r 2 >0.3, quality threshold >0.9, minor allele frequency >0.05, located at 500 kb up- or downstream of the four lead SNPs). For 6p21.32, a series of SNPs reaching P ≤1.0 × 10 −5 were in strong linkage disequilibrium (LD) with rs7194 (six SNPs: r 2 =0.997–0.998, P =1.51 × 10 −6 –3.99 × 10 −6 , Fig. 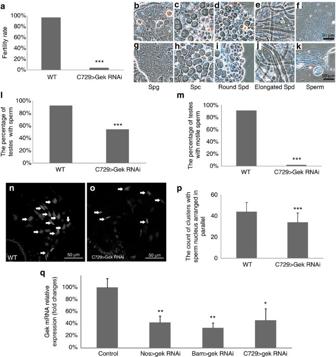Figure 2:Gekknockdown resulted in decreased male fertility. (a) A single male fertility test indicated that only 3.85% (n=52) ofc729>gek RNAimales are fertile compared with 96.9% (n=65) of wild-type flies at 28 °C. Each stage of the germ cells could be found in the testes of wild-type (b–f) andc729>gek RNAiflies (g–k) (spg, spermatogonia; spc, spermatocyte; round spd, round spermatid; elongated spd, elongated spermatid). Only 54.35% (n=46) ofc729>gek RNAitestes have morphologically mature sperm (l) and only 2.17% (n=46) ofc729>gek RNAitestes have motile sperm (m). Hoechst staining (white) showed decreased elongated spermatid bundles (arrows) in thec729>gek RNAitestis (n) compared with that in wild-type testis (o). (p) Quantification of elongated spermatid bundles in the wild-type testes (43.97±8.70,n=62) and thec729>gek RNAitestes (33.93±8.78,n=42).χ2tests were used for the comparisons of ratios, and Student’st-test was used for the comparison of the quantification of elongated spermatid bundles. Significant differences are indicated by (***P<0.001). (q) Efficiency ofgek RNAiknockdown evaluated by quantitative real-time PCR innos>gek RNAi,bam>gek RNAiandc729>gek RNAitestes (Student’st-test: *P<0.05; **P<0.01). Error bars represent the s.d. 1a and Supplementary Table 2 ). However, for 10q25.3, 6p12.2 and 1q42.13, we did not identify any untyped SNPs in high LD with the lead SNP reaching P ≤1.0 × 10 −5 ( Fig. 1b–d and Supplementary Table 2 ). Figure 1: Regional plot of the four identified lead SNPs. These SNPs are rs7194 at 6p21.32, rs7099208 at 10q25.3, rs13206743 at 6p12.2 and rs3000811 at 1q42.13. Additive models of logistic regression analyses were used to estimate the P values of association analyses in 981 NOA cases and 1,657 controls. The results (−log 10 P ) are shown for SNPs in the region flanking 500 kb on either side of the marker SNPs. The marker SNPs are shown in purple, and the r 2 values of the rest of the SNPs are indicated by different colours. The genes within the region of interest are annotated, with arrows indicating transcription direction. For each plot, the recombination rates (right y axes) of the region are shown according to their chromosomal positions ( x axis). Full size image Functional relevance of the Drosophila CDC42BPA orthologue Rs3000811 is located upstream of CDC42BPA (CDC42-binding protein kinase alpha), which has an orthologous gene named gek ( CG4012 ) in Drosophila . We then performed phenotypic analysis on its related gene in Drosophila using GAL4-driven UAS-short hairpin RNA system. We used nos-GAL4 , bam - GAL4 and c729-GAL4 to drive UAS-gek shRNA expression, and we found that nos>gek RNAi and bam>gek RNAi males were fertile and most c729 > gek RNAi males were infertile at 28 °C. To confirm the results, the single male fertility tests (one RNAi F1 male and three wild-type virgins in a tube) were conducted; all nos>gek RNAi ( n =50) and bam>gek RNAi ( n =50) males were fertile, and 96.15% ( n =52) of c729 > gek RNAi males were found to be completely infertile ( Fig. 2a ). Dissection results showed that ~\n54.35% ( n =46) of the c729>gek RNAi testes have each stage of germ cells ( Fig. 2b–k ), but only 2.17% have mature motile sperms ( Fig. 2l,m ). Nuclear dye staining also showed decreased elongated spermatid bundles in the c729>gek RNAi testes ( Fig. 2n–p ). Analysis of testicular gek mRNA expression showed significant suppression of gek in all three types of gek RNAi testes ( Fig. 2q ). For the other three SNPs (rs13206743, rs7194 and rs7099208) showing significant associations with NOA, we also analysed genes adjacent to these SNPs and did not find orthologous genes in Drosophila. Figure 2: Gek knockdown resulted in decreased male fertility. ( a ) A single male fertility test indicated that only 3.85% ( n =52) of c729 > gek RNAi males are fertile compared with 96.9% ( n =65) of wild-type flies at 28 °C. Each stage of the germ cells could be found in the testes of wild-type ( b – f ) and c729 > gek RNAi flies ( g – k ) (spg, spermatogonia; spc, spermatocyte; round spd, round spermatid; elongated spd, elongated spermatid). Only 54.35% ( n =46) of c729 > gek RNAi testes have morphologically mature sperm ( l ) and only 2.17% ( n =46) of c729 > gek RNAi testes have motile sperm ( m ). Hoechst staining (white) showed decreased elongated spermatid bundles (arrows) in the c729 > gek RNAi testis ( n ) compared with that in wild-type testis ( o ). ( p ) Quantification of elongated spermatid bundles in the wild-type testes (43.97±8.70, n =62) and the c729 > gek RNAi testes (33.93±8.78, n =42). χ 2 tests were used for the comparisons of ratios, and Student’s t -test was used for the comparison of the quantification of elongated spermatid bundles. Significant differences are indicated by (*** P <0.001). ( q ) Efficiency of gek RNAi knockdown evaluated by quantitative real-time PCR in nos>gek RNAi , bam>gek RNAi and c729>gek RNAi testes (Student’s t -test: * P <0.05; ** P <0.01). Error bars represent the s.d. Full size image During manuscript preparation, an independent GWAS of NOA in Han Chinese was conducted, involving 802 azoospermia cases (from Shandong province in Northern China based on Illumina OmniExpress BeadChip) and 1,863 controls (1,000 men from Shanghai in Southeastern China based on the Illumina OmniExpress BeadChip and 863 women from Shandong province based on the Affymetrix SNP Array 6.0) for discovery and a two-stage validation of 1,424 cases and 2,713 controls [8] . Interestingly, Zhao et al . [8] found four SNPs residing in a 144-kb genomic region at 6p22 around HLA-DRA (major histocompatibility complex, class II, DR alpha) to be associated with NOA risk at genome-wide significant level. These variants were suggested to mediate the response to testicular microenvironmental antigens and cause testicular azoospermia through autoimmune inflammatory responses [8] . The lead SNP rs7194 in the current study was close to and in high LD with the reported SNPs in the GWAS by Zhao et al . [8] (rs7194 is only 834 base pair apart from and in complete LD with rs7192). Supportive evidence was also reported in previous candidate gene-based studies in which HLA-DRB1 and -DQB1 alleles were found to be associated with NOA in Japanese patients [9] , [10] . A recently published study showed strong association of HLA-DPB1*04:01 with Japanese NOA [11] . To further assess the association of HLA region with NOA, we performed an imputation of classical HLA alleles in silico and analysed their associations with NOA in the samples of the initial GWAS stage. Nine alleles other than HLA-A and HLA-DPB1 alleles were associated with NOA, with P -values <0.05. All of the HLA alleles were in weak LD with rs7194, suggesting that the association of rs7194 with NOA risk may be independent from those classical HLA alleles ( Supplementary Table 3 ). However, these results need to be confirmed in large samples with experimental data. In expression quantitative trait locus (eQTL) analysis (Methods), rs7194 was significantly associated with the mRNA expression levels of a series of genes coding major histocompatibility complex (that is, HLA-DRA , HLA-DRB1 , HLA-DRB5 , HLA-C , HLA-DQA1 and HLA-DQB1 ) in lymphoblastoid cell lines or monocytes as a cis -acting element. In addition, rs7194 could influence the expression of C21orf127 and ERG (v-ets, erythroblastosis virus E26 oncogene homologue) as a trans -factor in monocytes. However, these results are preliminary and warrant further investigations. The SNP rs7099208 is within the last intron of FAM160B1 (family with sequence similarity 160, member B1) without known function and is 40 kb upstream of TRUB1 (TruB pseudouridine (psi) synthase family member 1) at 10q25.3. The TRUB1 products could be the human transfer RNA psi synthases, and its mRNA is reported to be widely expressed in various human tissues (especially heart, skeletal muscle and liver) [12] ; however, no data to date are available regarding its function in spermatogenesis. This lead SNP is also 210 kb upstream of ABLIM1 (actin-binding LIM protein 1). ABLIM1 was originally found in human retina and was postulated to regulate actin-dependent signalling [13] . In the testis, ABLIM1 may function in ectoplasmic specialization (ES), a testis-specific adherens junction. ES is known to be important for the connection between adjacent Sertoli cells and the formation of blood–testis barrier (BTB), as well as for the connection between Sertoli cells and elongating spermatids [14] . Moreover, silencing ABLIM1 in RPE1 cells leads to spontaneous ciliogenesis and significantly promotes cilia elongation [15] . Cilia and sperm flagella both have microtubule-based axoneme structure [16] , so ABLIM1 may also regulate flagellum development during spermatogenesis. We also identified associations with NOA for rs13206743, located 3 and 7 kb downstream of MIR133B and MIR206 , respectively. There is no correlative literature regarding the two microRNAs and spermatogenesis. The lead SNP is 34 kb upstream of interleukin (IL)-17A and 84 kb downstream of IL-17F . Studies have proven that testicular inflammatory disorders leading to impairment of spermatogenesis are the primary reasons for male infertility, and T helper cells play an essential role in this condition [17] , [18] , [19] . T helper 17 cells have been identified as a distinct lineage of CD4+ T cells and are characterized by the production of IL-17A, IL-17F and many other cytokines [20] , [21] . IL-17 is expressed in normal human testis at base line levels, suggesting that IL-17 may be involved in the maintenance of testicular immune privilege and spermatogenesis. However, an increased expression of IL-17A could be detected in azoospermic testis with chronic inflammation. Thus, overexpression of IL-17A could substantially damage the BTB and most likely destroy normal spermatogenesis and germ cells, which in turn could lead to azoospermia [22] . In addition, the SNP rs13206743 is ~\n65 kb upstream of PKHD1 (polycystic kidney and hepatic disease 1), which may serve as the PKHD1 promoter polymorphism. This gene is a disease-causing gene for autosomal recessive polycystic kidney disease [23] . Another lead SNP, rs3000811, lies in the 670 kb interval between CDC42BPA and ZNF678 (zinc-finger protein 678). We identified gek , which is an orthologous gene of CDC42BPA , as playing a phenotypic effect on male fertility in Drosophila . Our results showed that inhibiting expression of gek could lead to male infertility. C729-GAL4 is expressed in cyst cells, testis sheath and male accessory gland [24] , [25] . These findings suggest that the function of gek in soma is critical for male fertility. Although suppressing gek expression in germ cells with nos-GAL4 and bam-GAL4 does not affect male fertility, it is unclear whether gek is required in germ cells. Analysing null alleles of gek in the future is critical to solve the issues. According to these results, the function of CDC42BPA in human’s NOA is worth deep exploration. The protein encoded by CDC42BPA is a member of the serine/threonine protein kinase family and has been shown to bind CDC42. It may function as a CDC42 downstream effector mediating CDC42-induced peripheral actin formation and promoting cytoskeletal reorganization [26] . CDC42 has been reported to regulate cell adhesion and junction function through regulating filopodia formation, protein trafficking and actin cytoskeleton [27] . In mammalian testes, extensive junction restructuring occurs in the seminiferous epithelium at the Sertoli–Sertoli and Sertoli–germ cell interface to facilitate the different cellular events of spermatogenesis, such as mitosis, meiosis, spermiogenesis and spermiation [14] . Recent studies have shown that CDC42 and components of the polarity protein complexes work in concert with laminin fragments, cytokines and testosterone to regulate the events of cell–cell interactions in the seminiferous epithelium via a local autocrine-based regulatory loop known as the apical ES–BTB–basement membrane axis. This functional axis coordinates various cellular events during different stages of the seminiferous epithelium cycle of spermatogenesis [28] . In conclusion, we identified four susceptibility loci (6p21.32, 10q25.3, 6p12.2 and 1q42.13) of NOA in the Chinese population, extending our previous findings and advancing the understanding of NOA susceptibility. Study design This study was approved by the institutional review boards of each participating institution, including the institutional review board from Nanjing Medical University, Renji Hospital, Center of Reproductive Medicine, Tongji Medical College of Huazhong University of Science and Technology, Jinghua Hospital, the second hospital of Nanning, Shengjing Hospital, Nanjing Jinling Hospital, the Second Affiliated Hospital of Shandong University of Traditional Chinese Medicine, Peking University Shenzhen Hospital, Shandong Provincial Hospital and Huashan Hospital. We performed a four-stage case-control analysis. The GWAS phase included 981 NOA cases recruited from the Nanjing Center of Reproductive Medicine and 1,657 male controls from Nanjing. For validations, we enlarged the sample size by testing 1,144 NOA cases and 2,373 healthy male controls (745 cases and 1,444 controls from Southeastern China: Nanjing and Shanghai; 106 cases and 527 controls from Central China: Wuhan; and 293 cases and 402 controls from Northern China: Shenyang) for the first-stage validation, and additional 1,662 NOA cases and 2,535 healthy controls (559 cases and 534 controls from Southeastern China: Nanjing and Shanghai; 642 cases and 936 controls from Central China: Wuhan; 349 cases and 641 controls from Northern China: Shenyang; and 112 cases and 424 controls from Southern China: Nanning) for the second-stage validation. The 1,817 cases and 2,997 controls from the previous study were included in the first two validation studies. The 802 NOA cases and 1,001 male controls of the third-stage validation were from another independent GWAS of NOA in Han Chinese [8] . All infertile male subjects were genetically unrelated Han Chinese men and selected based on an andrological examination, including examination of medical history, physical examination, semen analysis, scrotal ultrasound, hormone analysis, karyotyping and Y-chromosome microdeletion screening. Those with a history of cryptorchidism, vascular trauma, orchitis, obstruction of the vas deferens, abnormalities in chromosome number or microdeletions of the azoospermia factor region on the Y chromosome were excluded from the study. Semen analysis for sperm concentration, motility and morphology was performed following World Health Organization (WHO) criteria (1999). Subjects with NOA had no detectable sperm in the ejaculate after evaluation of the centrifuged pellet. To differentiate from OA, only idiopathic azoospermic patients with small and soft testis, normal fructose and neutral alpha glucosidase in seminal plasma were included in the study. Those with a history of vasectomy were excluded. To ensure the reliability of the diagnosis, each individual was examined twice, and the absence of spermatozoa from both replicate samples was taken to indicate azoospermia. The GWAS control subjects were shared with the Nanjing Lung Cancer Study [29] , and all of these males had fathered one or more healthy children. In addition, the controls for the validation stage had fathered one or more healthy child. A 5-ml sample of whole blood was obtained from each participant as a source of genomic DNA for further genotyping analysis and all participants would complete the informed consent in written before taking part in this research. SNP selection and genotyping for validation Because the control group was shared with the Nanjing Lung Cancer Study, the NOA cases were compared with two control groups separately or in combination with the discovery phase to avoid potential effects from lung cancer [7] . We selected SNPs meeting the following criteria for the first-stage validation: (i) SNPs had 1.0 × 10 −7 < P ≤1.0 × 10 −5 in the comparison between 981 NOA cases and 1,657 controls and had a consistent association at P ≤1.0 × 10 −2 when the NOA cases were compared separately with the healthy male controls and the male lung cancer cases in additive models of logistic regression analyses; (ii) not located in the same chromosome region/gene of SNPs reported in our previous GWAS study; (iii) SNPs had clear genotyping clusters; and (iv) only the SNP with the lowest P value was selected when multiple SNPs were observed in a strong LD ( r 2 ⩾ 0.8). A total of 77 SNPs met these criteria ( Supplementary Data 1 ). Significantly associated SNPs ( P <0.05) were further genotyped in validation samples. Genotyping analyses were performed using the middle-throughput TaqMan OpenArray Genotyping Platform (Applied Biosystems, USA), the iPLEX Sequenom MassARRAY platform (Sequenom, CA, USA) and the TaqMan allelic discrimination Assay (Applied Biosystems). The primers and probes are available on request. The primers of nine SNPs using TaqMan allelic discrimination Assay to perform genotyping were provided in Supplementary Table 4 . A series of methods were used to control the quality of genotyping: (i) case and control samples were mixed on each plate; (ii) genotyping was performed without knowing the case or control status; (iii) two water controls were used in each plate as blank controls; and (iv) five per cent of the samples were randomly selected for repeat genotyping. Statistical analysis The association analysis was performed using an additive model in a logistic regression analysis using the PLINK 1.07 program ( http://pngu.mgh.harvard.edu/~purcell/plink/ ). Meta-analysis was performed in a combined analysis, and a random-effects model was used when heterogeneity between studies exists, that is, P value for heterogeneity test is <0.05; otherwise, a fixed-effect model was used. We used MACH 1.0 software ( http://www.sph.umich.edu/csg/abecasis/MACH/index.html/ ) to impute ungenotyped SNPs using LD information from the hg18/1,000 Genomes Project database (CHB+JPT as a reference set; June 2010 release). The chromosome region was plotted using the LocusZoom 1.1 program ( http://csg.sph.umich.edu/locuszoom/ ). Other analyses were performed with R software (version 2.11.1; The R Foundation for Statistical Computing; http://www.cran.r-project.org/ ). HLA alleles were predicted from dense SNP genotypes using the R software package, HIBAG ( http://cran.r-project.org/web/packages/HIBAG/index.html ). eQTL analysis We performed eQTLs analysis using the University of Chicago eQTL Browser ( http://eqtl.uchicago.edu/cgi-bin/gbrowse/eqtl/ ), which contains significant eQTLs identified in recent studies across multiple cell lines and populations. Fly strains and genetics The fly strains were obtained from the Bloominton Stock Center. Flies were cultured with standard culture medium. To enhance the knockdown efficiency, culture tubes were put into 28 °C incubators after egg laying. The male fertility tests were performed at room temperature. For single male fertility test, freshly hatched single males were crossed to multiple virgin Canton S flies and the presence of progeny (including larvae, pupae and adults) was scored after 10–15 days. Testis analysis Testis squashes were prepared in TB1 buffer (7 mM K 2 HPO 4 , 7 mM KH 2 PO 4 [pH 6.7], 80 mM KCl, 16 mM NaCl, 5 mM MgCl 2 , 1% PEG-6000) according to previous report [30] . Phase contrast light micrographs were taken, and mature and motile sperm were observed under a microscope. To count the elongated spermatid bundles, testes from freshly hatched males were dissected, fixed and stained with Hoechst 33342 dye. Confocal image stacks were taken, and elongated spermatid bundles were counted. Gek mRNA expression in adult testes was analysed by quantitative real-time PCR with 18s mRNA as reference. The primers used were as follows, gek (forward), 5′-CGAAAGGGACTTCCGAGCAT-3′; gek (reverse), 5′-TCGGAGTTTGCATCCACTTGT-3′; 18s RNA (forward), 5′-TGGTTTCCGGCAAGCTTCAA-3′; 18s RNA (reverse), 5′-ACTTCTTGAATCCGGTGGGC-3′. How to cite this article: Hu, Z. et al . Association analysis identifies new risk loci for non-obstructive azoospermia in Chinese men. Nat. Commun. 5:3857 doi: 10.1038/ncomms4857 (2014).